Engineering particle trajectories in microfluidic flows using particle shape Recent advances in microfluidic technologies have created a demand for techniques to control the motion of flowing microparticles. Here we consider how the shape and geometric confinement of a rigid microparticle can be tailored for ‘self-steering’ under external flow. We find that an asymmetric particle, weakly confined in one direction and strongly confined in another, will align with the flow and focus to the channel centreline. Experimentally and theoretically, we isolate three viscous hydrodynamic mechanisms that contribute to particle dynamics. Through their combined effects, a particle is stably attracted to the channel centreline, effectively behaving as a damped oscillator. We demonstrate the use of self-steering particles for microfluidic device applications, eliminating the need for external forces or sheath flows. In slow viscous flows, suspended particles are coupled by the flow disturbances they create in the surrounding fluid. These hydrodynamic interactions (HIs) can drive spatial organization of a microparticle or system of microparticles in geometric confinement. Specific examples include the cross-stream migration of a single polymer near a wall [1] , the clustering of red blood cells in a tube [2] and the crystallization of rigid spheres with finite inertia in a square channel [3] , [4] . Both practical and theoretical considerations motivate interest in hydrodynamic ‘self-steering’ (of a single particle) and self-organization (of multiple interacting particles). In microfluidic devices, control over particle position allows the high throughput performance of operations on individual flowing objects, for example, in on-chip cytometry [5] and multiplexed assays with functionalized particles [6] . Although particles can be directly positioned with external fields or sheath flows [6] , [7] , these methods can require cumbersome apparatus or complex channel structure. An elegant alternative is to tailor particle and channel design for self-steering or self-organization. Moreover, if the self-steered position of an object depends on a certain property of the object, a heterogeneous suspension can be separated by that property. For instance, both the stiffness [8] and shape [9] of blood components are of interest for microfluidic separations. From a theoretical perspective, a unifying framework for non-equilibrium self-organization and self-steering is highly sought after [10] . Specific mechanisms for cross-streamline migration and focusing in channel flow have been extensively investigated for Brownian [11] , inertial [3] , [4] and deformable [1] , [2] particles. In these cases, migration arises from the interplay of viscous hydrodynamics near a channel boundary and another physical effect that breaks the reversibility of viscous flow. Conceptually, it seems difficult to reconcile self-organization and self-steering, in which any initial state will evolve towards one of a limited set of dynamical attractors, and reversibility, which requires particle behaviour to make no distinction between two possible directions of time. Confining boundaries can change the spatial decay and even the tensorial structure of HIs. Interactions take a unique form when the typical particle size is comparable to the height of a confining slit, such that the particles are constrained to ‘quasi-two-dimensional’ (q2D) motion ( Fig. 1a ). The tightly confined particles experience strong friction from the confining plates, and will therefore lag a pressure-driven external flow. In lagging the flow, the particles create flow disturbances with a characteristic dipolar structure: moving upstream relative to the fluid, particles push fluid away from their upstream edges and draw fluid into their downstream edges. This far-field flow disturbance, the ‘source dipole’, is given by the conservation and transport of fluid mass, and decays as 1/ r 2 (refs 12 , 13 ). In contrast, the leading order far-field disturbance in bulk (three-dimensional) fluid, the ‘Stokeslet’, is given by the conservation and transport of momentum, and decays as 1/ r . The difference between bulk and q2D arises because of the confining plates, which, by exerting friction on the fluid, dissipate momentum and screen its long-range transport, leaving only mass to determine the far-field disturbance. 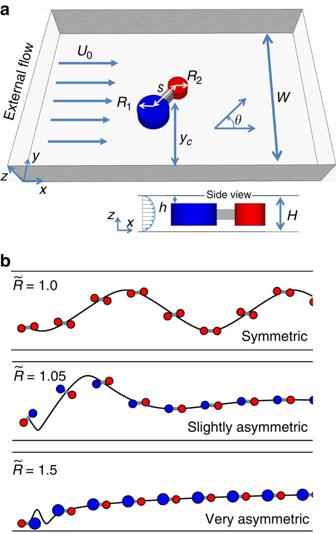Figure 1: Model particle geometry and behaviours. (a) Schematic diagram of the model system. A particle comprising two rigidly connected discs is confined in a thin microchannel and driven by an external flow. (b) Behaviours obtained as particle asymmetry is varied. A symmetric particle oscillates between side walls. When the symmetry is slightly broken, this oscillation is damped and the particle aligns with the flow as it focuses to the centreline. A very asymmetric particle is ‘overdamped’, and rapidly aligns before slowly focusing. The trajectories inbwere obtained numerically for the parameters given in the caption ofFig. 5b. Thexaxes are scaled by a factor of 1/40 to show the full range of particle behaviours. Figure 1: Model particle geometry and behaviours. ( a ) Schematic diagram of the model system. A particle comprising two rigidly connected discs is confined in a thin microchannel and driven by an external flow. ( b ) Behaviours obtained as particle asymmetry is varied. A symmetric particle oscillates between side walls. When the symmetry is slightly broken, this oscillation is damped and the particle aligns with the flow as it focuses to the centreline. A very asymmetric particle is ‘overdamped’, and rapidly aligns before slowly focusing. The trajectories in b were obtained numerically for the parameters given in the caption of Fig. 5b . The x axes are scaled by a factor of 1/40 to show the full range of particle behaviours. Full size image These unique features of the dipolar flow disturbance allow the realization of ‘flowing crystals’ with novel collective modes [14] , [15] , [16] , [17] . These are configurations of particles that maintain spatial order as they are advected by an external flow. They are marginally stable: the amplitude of a collective mode neither grows nor decays in time. Consequently, realization of crystals is limited by initial configuration, and they are sensitive to break-up via nonlinear instabilities and channel defects. A natural question is how to introduce an effective attraction to the crystalline states, causing particles to assemble from disorder, and providing a ‘restoring force’ against perturbations. One indication is provided by a recent study which demonstrated stable pairing of droplets via the higher flow disturbance multipoles induced by shape deformation [18] . This finding suggests a key role for particle shape in achieving self-steering and self-organization. In this study, we combine theoretical and experimental approaches to investigate how particle shape can be tailored to induce self-steering under flow in q2D microchannels. Our main finding is that a single rigid, asymmetric particle will spontaneously align with the external flow and focus to the channel centreline. This self-steering can be tuned via channel and particle geometry. Moreover, it is time reversible; to our knowledge, all previous instances of hydrodynamic self-steering have been irreversible. Through a simple theoretical model, confirmed by experiments, we demonstrate how assembly arises from the interplay of three viscous effects: rotation and cross-streamline migration, via a particle’s hydrodynamic self-interaction, and rotation via a particle’s interaction with hydrodynamic images. Each effect has an analogue in bulk sedimentation, but not in bulk channel flow. We demonstrate application of these findings in a device setting. Finally, we discuss their implications for the design of self-organizing ‘swarms’ of interacting particles. Model system and governing parameters We consider a simple model geometry that captures the generic effects of asymmetry. A particle comprises two discs of radius R 1 and R 2 , with R 1 ≥ R 2 , which are rigidly connected with distance s between their centres. It is confined in a shallow channel of height H in the z -direction and width W in y . Two lubricating gaps of height h separate each of the discs from the confining walls in z ( Fig. 1a ). There is a pressure-driven flow in x with a parabolic profile in z and an approximately uniform depth-averaged velocity U 0 (Hele-Shaw flow). In the absence of inertia, the governing dimensionless parameters are geometric: , , , and (ref. 19 ). We define dimensionless time as . The instantaneous particle configuration is defined by the location in y of the midpoint between disc centres, y c ≡ ( y 1 + y 2 )/2, and angle θ between the external flow and the particle axis, shown in Fig. 1a . Owing to translational symmetry, the position in the flow direction x c ≡ ( x 1 + x 2 )/2 does not affect particle dynamics. We describe the theoretical model and the experimental method in detail in the Methods section. In the model, we write a force balance equation for each disc. Each disc experiences drag from the local flow and friction from the confining plates, as detailed analytically in Supplementary Note 1 , in addition to a rigid constraint force. The local flow at each disc is determined self-consistently as the external flow plus contributions from the other disc and the discs’ hydrodynamic images. The system of images, previously obtained in Uspal and Doyle [20] and presented in Supplementary Note 2 , imposes a no mass flux boundary condition on the confining side walls. In the experiments, we use continuous flow lithography (CFL) to fabricate particles with desired shape and initial configuration in situ under q2D channel flow. Hydrodynamic self-interaction As the first step in building a complete picture of particle dynamics, we neglect the effect of side walls, isolating a particle’s self-interaction. For an identical pair of discs, the interaction is symmetric: disc 1 pushes on disc 2 just as much as disc 2 pushes on disc 1 ( Fig. 2a ). The interaction cannot lead to relative motion of the discs, including rotation of the entire particle [21] . However, when θ ≠0° and θ ≠90°, it introduces a component to the particle velocity perpendicular to the direction of the external flow [20] . When 0°< θ <90°, the particle migrates in the direction of decreasing y ; when 90°< θ <180°, it migrates with increasing y . This ‘lateral drift’, occurring for both symmetric and asymmetric particles, also occurs for a rod or pair of spheres sedimenting in bulk. 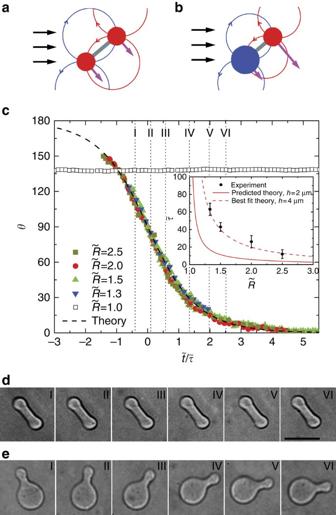Figure 2: Self-alignment of a particle in unbounded q2D. (a) Illustration of the self-interaction of a symmetric particle. A disc’s vector shows the component of the flow disturbance from the other disc in, the direction of increasingθ. The vectors are identical: there is no rotation of the particle. (b) When the two discs have different radii, the particle aligns with the flow. (c) Experimental angle vs time for variouswith,and. We scale the data for eachby a fitted, collapsing all data onto a universal curve predicted by theory. (inset) The dependence of the experimental timescaleson, along with a theoretical curve for the same parameters (solid) and a theoretical curve withadjusted for best fit (dashed). Each experimental data point is an average of timescales measured for nine individual particles; error bars indicate the standard deviation. (d) Snapshots of a symmetric particle at various times, matched to the times inc. Scale bar, 100 μm. (e) Snapshots forat the same times as ind. Figure 2: Self-alignment of a particle in unbounded q2D. ( a ) Illustration of the self-interaction of a symmetric particle. A disc’s vector shows the component of the flow disturbance from the other disc in , the direction of increasing θ . The vectors are identical: there is no rotation of the particle. ( b ) When the two discs have different radii, the particle aligns with the flow. ( c ) Experimental angle vs time for various with , and . We scale the data for each by a fitted , collapsing all data onto a universal curve predicted by theory. (inset) The dependence of the experimental timescales on , along with a theoretical curve for the same parameters (solid) and a theoretical curve with adjusted for best fit (dashed). Each experimental data point is an average of timescales measured for nine individual particles; error bars indicate the standard deviation. ( d ) Snapshots of a symmetric particle at various times, matched to the times in c . Scale bar, 100 μm. ( e ) Snapshots for at the same times as in d . Full size image When the discs are dissimilar, the particle aligns itself with the external flow, such that the larger disc is upstream of the smaller disc ( Fig. 2b ). The principal cause of self-alignment is that one disc is hydrodynamically stronger than the other: in q2D, the magnitude of the dipolar flow disturbance created by a disc scales as the disc area. In Supplementary Note 3 , we derive an exact expression for θ as a function of time. Taking t =0 when θ =90°, we obtain , where the timescale depends on particle geometry. Notably, it diverges for . We recover these predictions experimentally. We polymerize particles with various and measure how θ evolves with . We fit a timescale to the data of each . When θ is plotted against , all data collapses onto a universal curve ( Fig. 2c ). We leave the data for unscaled; for this singular case, the particle maintains its initial angle. The curve asymptotes to θ =0° and θ =180°, and is manifestly time reversible. In the inset of Fig. 2c , we plot the dependence of the experimental timescales on alongside a theoretical curve predicted for the same parameters. The theoretical and experimental timescales have the same order of magnitude and the same trend with . Moreover, by adjusting , we generate a theoretical curve with good fit to the data. The effect of the physics our model neglects is simply to renormalize . Hydrodynamic self-orientation has not been observed for a rigid particle in bulk channel flow. Bretherton considered bodies with axial and fore-aft symmetry in slow unidirectional shear flows, which include pressure-driven bulk channel flows. He found that nearly all particles tumble in Jeffery orbits with no equilibrium orientation and no cross-streamline migration, except for certain ‘extreme’, high aspect ratio shapes [22] . To our knowledge, these shapes have not been realized experimentally. Subsequently, flow-driven doublets of unequal spheres, analogous to the dumbbells we consider, were studied by Nir and Acrivos [23] and Adler [24] . These also tumble with no net migration. However, self-alignment has recently been predicted for asymmetric objects in bulk sedimentation, with a dynamical equation similar to ours when the object is initially oriented in a vertical plane [25] . Effect of hydrodynamic images Having isolated a particle’s self-interaction, we consider how it combines with image interactions to produce the behaviours of Fig. 1b . Consider the symmetric particle in Fig. 3 . To leading order, the translation in y arises from self-interaction. The chief effect of the images is to rotate the particle. The particle in Fig. 3 begins by migrating towards the lower wall. It is rotated into θ =0°, for which the lateral velocity is zero. This configuration is an extremum of the oscillation. The particle is rotated further and migrates away from the wall. The mirror symmetry of the particle at the extremum ensures that the outgoing trajectory is mirror symmetric with the incoming trajectory. After crossing the centreline, the particle will reflect from the upper wall. Moreover, an oscillation with a θ =90° extremum can be produced with a different initial condition. Again, we can find an analogue in bulk sedimentation; a rod falling between vertical walls will oscillate between them with θ =0° and θ =90° modes of reflection [26] . Numerically, we construct a phase portrait for a symmetric particle ( Fig. 5b ), showing trajectories in the space of particle configurations ( y c , θ ). Owing to the properties of viscous flow, the spatial configuration of a particle completely specifies the state of the system. We find that there are marginally stable fixed points at ( y c , θ )=( W /2,0°) and ( y c , θ )=( W /2,90°), each of which is associated with a continuous family of periodic orbits. 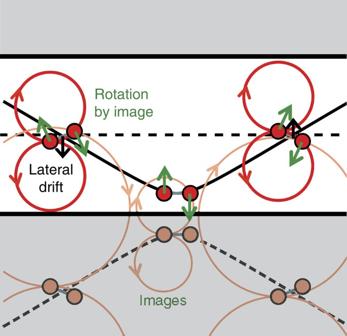Figure 3: Oscillation of a symmetric particle. A symmetric particle oscillates via the combined effects of HI with itself and with its own images. Self-interaction leads to cross-streamline migration (‘lateral drift’) when the particle angleθ≠0° andθ≠90°. The images rotate the particle. Figure 3: Oscillation of a symmetric particle. A symmetric particle oscillates via the combined effects of HI with itself and with its own images. Self-interaction leads to cross-streamline migration (‘lateral drift’) when the particle angle θ ≠0° and θ ≠90°. The images rotate the particle. 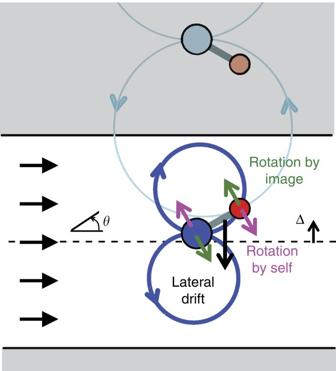Figure 4: Linearized model of an asymmetric particle. Rotation by the images is opposed by self-alignment. The particle drifts in theydirection whenθis displaced from the equilibrium valueθ=0°. The lateral displacement Δ is defined as Δ≡yc−W/2. Full size image Figure 4: Linearized model of an asymmetric particle. Rotation by the images is opposed by self-alignment. The particle drifts in the y direction when θ is displaced from the equilibrium value θ =0°. The lateral displacement Δ is defined as Δ≡ y c − W /2. 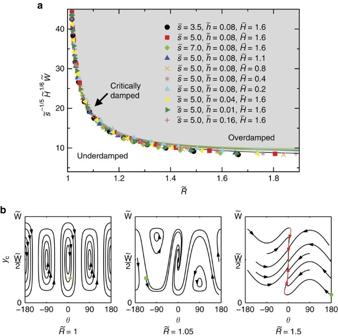Figure 5: Phase diagram and portraits. (a) Phase diagram showing the critical boundary that separates the underdamped and overdamped regimes. The symbols are points on the boundary obtained numerically for various parameters. The solid lines, matched by colour to the symbols, are theoretical curves for the same parameters. The numerical data and theoretical curves collapse onto one universal boundary. (b) Portraits showing particle trajectories in the phase space (yc,θ). Portraits were obtained numerically for,,and. Arrows give direction of motion in phase space. Dots identify the trajectories shown inFig. 1b. Full size image Figure 5: Phase diagram and portraits. ( a ) Phase diagram showing the critical boundary that separates the underdamped and overdamped regimes. The symbols are points on the boundary obtained numerically for various parameters. The solid lines, matched by colour to the symbols, are theoretical curves for the same parameters. The numerical data and theoretical curves collapse onto one universal boundary. ( b ) Portraits showing particle trajectories in the phase space ( y c , θ ). Portraits were obtained numerically for , , and . Arrows give direction of motion in phase space. Dots identify the trajectories shown in Fig. 1b . Full size image For an asymmetric particle, self-alignment changes the fixed point ( y c , θ )=( W /2,0°) into an attractor, as we demonstrate with a linearized model ( Fig. 4 ). We define Δ ≡ y c − W /2, and model lateral drift as , where a >0 depends on the dimensionless parameters. We model the rotational dynamics by , with coefficients b >0 and c ≥ 0 that, respectively, capture the strength of the images and self-alignment. When the particle is displaced from the centreline (Δ≠0), the effect of the images is to rotate the particle away from θ =0°, which is opposed by self-alignment. These equations can be combined into . Without self-alignment ( c =0), the particle oscillates around the fixed point. When c ≠0, the particle is attracted to the fixed point via either a decaying oscillation or an ‘overdamped’ approach. These regimes are separated by a critical boundary in parameter space . Numerically, we construct a boundary by finding the critical as a function of for various sets of the parameters , and , as described in Supplementary Note 4 . We also obtain expressions for a , b and c via heuristic arguments, yielding a function that fits the numerical data for each individual parameter set ( Supplementary Fig. S1 ). We collapse the numerical data and theoretical curves with the empirically fitted scaling in Fig. 5a , exposing the universal shape of the curve. This phase diagram can guide the design and optimization of self-steering particles. For a given set of parameters , and , focusing occurs over the shortest streamwise travel distance at , as the analogy with a ‘critically damped’ oscillator suggests ( Supplementary Note 5 and Supplementary Fig. S2 ). The critical boundary occurs when the timescale for self-alignment is comparable to the timescale for a particle to migrate across the channel width. Along the boundary, decreasing while increasing or decreasing is an effective design strategy to reduce streamwise travel distance by decreasing lateral migration distance and enhancing self-alignment. Strikingly, the diagram does not depend on , the dimensionless lubricating gap thickness, which can be independently tuned. Decreasing slows down the particles, strengthening HIs and reducing the travel distance for focusing. Having considered small displacements from ( y c , θ )=( W /2,0°), we construct phase portraits for and ( Fig. 5b ). The slightly asymmetric particle approaches ( y c , θ )=( W /2,0°) via a decaying oscillation, but there are marginally stable fixed points with θ =±90°. These ‘bouncing states’ are due to the interaction of a particle with a nearby image ( Supplementary Note 6 and Supplementary Fig. S3 ). For , any point in the phase space is along a trajectory connecting the unstable fixed point ( y c , θ )=( W /2,180°) with the stable fixed point. For a highly asymmetric particle, there is a separation of timescales between rapid self-alignment and slow lateral focusing. This separation can be seen in the convergence of all trajectories to a slow manifold, outlined in red. As the attractor is asymptotic and accompanied by a repeller, it is compatible with reversibility: if the flow is reversed, the fixed points exchange stability, and a particle retraces its trajectory in phase space, attracted to the other fixed point. We explicitly demonstrate reversibility in Supplementary Fig. S4 and Supplementary Note 7 . Our complete theoretical picture predicts a wide range of experimental observations involving both the channel side walls and particle self-interaction. We first consider three particle trajectories in individual detail. 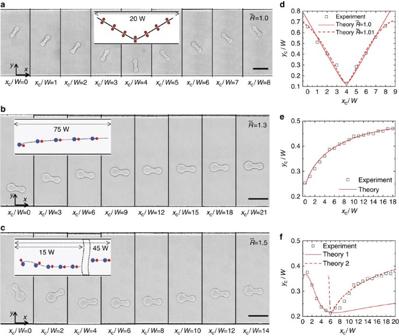Figure 6: Individual particle trajectories. Scale bars, 100 μm. (a) Experimental montage showing reflection of a symmetric particle. The corresponding theoretical trajectory is shown in the inset. (b) A strongly asymmetric particle withθ=−10° focuses to the centreline. (c) A strongly asymmetric particle with a large initial angle aligns and then focuses to the centreline. (d) Position data for the trajectory ina. The theoretical trajectory forwas scaled inxby a factor of 0.475. A theoretical curve with, for which the rescaling is 0.4, better captures the curvature of the data. (e) For the particle inb, the rescaling is 0.15. (f) For the two timescale process ofc, different rescalings of 3 and 0.1 are required to capture the initial and steady dynamics. For all trajectories,,and. Figure 6a and Supplementary Movie 1 show an experimental montage in which a symmetric particle is reflected from a side wall. We obtain qualitative agreement with the theoretical trajectory generated for the same parameters and initial conditions as the experiment, shown in the inset. The trajectory is shown quantitatively in Fig. 6d . The theoretical prediction can be fitted to the experimental data if it is rescaled in x . If we relax the assumption of perfect symmetry and take , the resulting theoretical curve better captures the curvature of the data. This asymmetry corresponds to a difference in radii of ~0.2 μm, within the uncertainty of CFL ( Supplementary Methods and Supplementary Fig. S5 ). In Fig. 6b and Supplementary Movie 2 , an asymmetric particle with polymerized with θ =−10° focuses to the channel centreline. Good agreement between theory and experiment is obtained upon rescaling. This initial condition is near the slow manifold for overdamped dynamics. For a particle with θ =135°, we obtain the predicted two timescale process of initial reorientation followed by slow focusing ( Fig. 6c ). This difference in timescales is manifested in different rescalings needed to fit theory to data for the initial dynamics, dominated by self-interaction and for focusing, in which the images are important. Figure 6: Individual particle trajectories. Scale bars, 100 μm. ( a ) Experimental montage showing reflection of a symmetric particle. The corresponding theoretical trajectory is shown in the inset. ( b ) A strongly asymmetric particle with θ =−10° focuses to the centreline. ( c ) A strongly asymmetric particle with a large initial angle aligns and then focuses to the centreline. ( d ) Position data for the trajectory in a . The theoretical trajectory for was scaled in x by a factor of 0.475. A theoretical curve with , for which the rescaling is 0.4, better captures the curvature of the data. ( e ) For the particle in b , the rescaling is 0.15. ( f ) For the two timescale process of c , different rescalings of 3 and 0.1 are required to capture the initial and steady dynamics. For all trajectories, , and . Full size image Finally, we apply the insights developed in this manuscript to engineer a practical microfluidic system with self-focusing particles. We can thereby build a statistical picture of particle dynamics from hundreds of trajectories. We fabricate asymmetric and symmetric fluorescent particles in a synthesis channel and collect them from the channel outlet in an Eppendorf tube containing a common buffer. After rigorously washing the particles by successive steps of gentle centrifugation and decanting, we resuspend the particles in approximately density matched solvent at the desired concentration and flow the suspension through a detection channel. In the detection channel, we measure the transverse position y c of each flowing particle near the inlet and the outlet with fluorescence microscopy. The results are shown in Fig. 7 and Supplementary Movies 3 and 4 . Starting from a broad and essentially random distribution of transverse positions, most asymmetric particles focus to the centreline. The finite width of the central peak is due to the finite length of the channel; with a longer channel, it would be narrower. The two side peaks are possibly due to the high shear rate in the boundary layer near the walls. In contrast, the symmetric particles remain unfocused. These results demonstrate both ‘self-steering’ for particle-based assays, as the asymmetric particles are focused and aligned for interrogation, and simple shape-based separation, as the centreline is enriched with asymmetric particles at the outlet. We also observe that a small fraction of both the symmetric and asymmetric particles (<12%) remain close to the walls at all times. 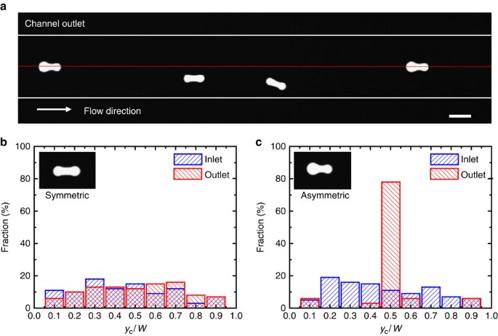Figure 7: Statistics of particles in a flow-through device. (a) Fluorescence microscopy image of symmetric and asymmetric particles flowing in a channel. The asymmetric particles focus to the centreline (red). The white lines indicate the channel side walls. Scale bar, 100 μm. (b) Distributions of transverse positions for symmetric particles () measured near the inlet (blue, left hatching) and outlet (red, right hatching). Both distributions are nearly uniform across the channel width. (c) Distributions of transverse positions for the asymmetric particles (). The particles begin nearly uniformly distributed at the inlet. Most focus to the centreline near the outlet. Statistics are gathered from over 300 symmetric and 300 asymmetric particle trajectories. Figure 7: Statistics of particles in a flow-through device. ( a ) Fluorescence microscopy image of symmetric and asymmetric particles flowing in a channel. The asymmetric particles focus to the centreline (red). The white lines indicate the channel side walls. Scale bar, 100 μm. ( b ) Distributions of transverse positions for symmetric particles ( ) measured near the inlet (blue, left hatching) and outlet (red, right hatching). Both distributions are nearly uniform across the channel width. ( c ) Distributions of transverse positions for the asymmetric particles ( ). The particles begin nearly uniformly distributed at the inlet. Most focus to the centreline near the outlet. Statistics are gathered from over 300 symmetric and 300 asymmetric particle trajectories. Full size image Experimentally and theoretically, we have shown that asymmetric particles flowing in a q2D channel self-steer − align with the flow and focus to the centreline − while symmetric particles oscillate between side walls. Via an analogy to a damped oscillator, we isolated three contributing hydrodynamic mechanisms and exhaustively revealed the dependence of the dynamics on the governing parameters, recovering the critical boundary between underdamped and overdamped regimes. Experiments and theory agree qualitatively and semiquantitatively. Uniquely, focusing in q2D channel flow requires no physics beyond viscous hydrodynamics. In contrast, an axisymmetric rigid particle in bulk channel flow tumbles in a modified Jeffery orbit with no net migration [22] , [23] , [24] , [27] . Chiral particles migrate across streamlines, but do not focus [28] , possibly because they have no equilibrium orientation. For the same reason, we suspect that curved fibres, recently predicted to migrate [29] , will not focus either. On the other hand, we found intriguing connections between q2D channel flow and bulk sedimentation, which may be due to a common feature: to leading order, the singularities that couple particles maintain fixed orientation. In sedimentation, gravity introduces point forces oriented in the vertical direction; in q2D channel flow, dipoles are approximately oriented upstream. In contrast, consider an axisymmetric rigid particle in bulk and driven by flow. Owing to the inextensibility of the particle, it creates a force dipole (pair of Stokeslets) that disturbs the flow if the particle is subject to a straining field, such as Poiseuille flow. The orientation and sign of this dipole depends on the particle orientation. Consequently, the periodicity of a Jeffery orbit entails that the force dipole averages out, as the particle equally samples the axes of extension and compression. With zero net force dipole, no net lift is produced by images introduced by confining boundaries. We have also shown that self-steering does not require irreversible physics, contrary to common intuition. Reversibility is not violated if an asymptotic attractor in phase space is accompanied by an asymptotic repeller. Our findings open a new direction for passive manipulation of particles flowing in microdevices: trajectories can be engineered via particle shape and confinement. We demonstrated that dilute suspensions of asymmetric particles entering a q2D channel in a random spatial distribution will exit in an aligned and focused stream if the channel is sufficiently long. Symmetric particles, on the other hand, show no focusing effect. A lab-on-a-chip system that applies these findings will not require external forces or sheath flows to position particles, simplifying device design, manufacture and use. In the same demonstration, we also performed a shape-based separation, enriching the centreline with asymmetric particles. Insights gained from this demonstration suggest future applications. We may be able to polymerize bifunctional particles containing a fluorescent code on the downstream edge of the particle and containing biomolecular capture probes such as DNA or antibodies in the upstream edge of the particle. These can be used for bioassays, harnessing previously shown advantages of using hydrogel particles for biosensing [30] . It is important to note that the particles considered here always align in the same direction, in contrast with particles aligned with sheath flows, such as in flow cytometry. Our results also provide the foundation for study of q2D systems in which particle–particle interactions are important, including multiparticle clusters and concentrated suspensions. In such systems, the flowing crystalline states discussed in the introduction are possible. In preliminary numerical work, clusters assemble into the one-dimensional crystalline states described in Uspal and Doyle [15] , in which particles are ordered in the lateral direction, and suspensions self-organize into two-dimensional crystals. We anticipate that our mechanistic insights into single particle dynamics will generalize to these ‘swarms’. Numerical model We assume the creeping flow or zero Reynolds number limit. The velocity of disc i , , is given by a force balance: where U ( r i ) is the depth-averaged velocity at the disc position r i =( x i , y i ), γ c ≡ 12 μ / H , μ is the fluid viscosity, which ultimately drops out of the equations, and F i is a force of rigid constraint if disc i is connected to another disc. ζ i is a drag coefficient, derived in Supplementary Note 1 . We assume simple shear in the lubricating gaps, so that the disc friction coefficient γ p =2 μ / h . Significantly, γ p > γ c , so that a disc will lag its local flow field, creating a dipolar disturbance. For a free (non-connected) disc, this lag has a simple expression: as F i =0, equation (1) can be rearranged as . α i characterizes the mobility of disc i , with 0< α i <1. In Supplementary Fig. S6 , we demonstrate good agreement of this simple model with the more detailed analysis of Halpern and Secomb [19] . The only free parameters are , , , and , defined above. A rigid constraint k between discs i and j is associated with a constraint equation and a force F ( k ) , where r ij ≡ r i − r j . In our disc-rod model of a dumbbell particle, the rigid constraint and the four disc force balance equations realize one torque balance and two force balance conditions. To simplify the analysis, we neglect the effects of lubrication forces and the rotation of individual discs. In Supplementary Note 8 and Supplementary Figs S7 and S8 , we show that including disc rotations would improve the quantitative accuracy of our model, but not change our qualitative findings. The local flow field at disc i is determined through an implicit equation where G ( ij ) ( r ij , r j ) is a tensor containing the leading order, far-field contribution of disc j to the local field at i . This tensor, given in Supplementary Note 2 , includes the effect of the hydrodynamic images needed to impose boundary conditions at the side walls. The hydrodynamic strength of disc j is characterized by a quantity that scales G ( ij ) . The constraint equations and equations (1) and (2) can be arranged into matrix form AU p = B , where U p is a vector containing all 2 N disc velocities, 2 N local fields and n constraint forces. We consider a single particle, so that N =2 and n =1. A is a matrix constructed from disc interactions, and B collects terms involving U 0 . This system can be solved and integrated numerically. Continuous flow lithography The complete experimental setup is depicted in Supplementary Fig. S9 . Particles with predefined geometries are synthesized in situ at the desired initial position and orientation using CFL, described in detail in Dendukuri et al. [31] In brief, an acrylate oligomer (poly(ethylene glycol) diacrylate) mixed with a photoinitiator is pumped through the poly(dimethylsiloxane) channel depicted in Fig. 1a using external pressure. The channel is mounted on an inverted microscope. Particles are polymerized with short pulses of ultraviolet light (50 ms for Fig. 2 and 100 ms for Fig. 6 .) The geometry of the particle in the xy plane is imposed by a lithographic mask placed between the microscope objective and the ultraviolet source. The height of the particle inside the channel is dictated by the ultraviolet exposure time [32] . Importantly, the well-known oxygen inhibition effect in the CFL method [31] , [32] provides uniformly thin, unpolymerized, lubricating layers between the microparticle and the top and bottom poly(dimethylsiloxane) walls. Particle height can be measured in the channel outlet, where some flip to their sides, as shown in Supplementary Fig. S10 . A complete list of synthesized particle geometries is provided in Supplementary Table S1 . Channels are 30 μm in depth, 500 μm in width and 2.4 cm in length. Using the hydraulic diameter 2 HW /( H + W ) as a length scale, 55 cp as the prepolymer viscosity, 50 μm s −1 as a typical flow speed and 1.12 × 10 3 kg m −3 as the prepolymer density, a typical Reynolds number is Re=6 × 10 −5 . Inertial effects are therefore negligible. As the particles move along the channel, the microscope stage is translated by a homemade linear motor, ensuring that the particles remain in the field of view. Movies of particle trajectories are recorded using a CCD camera and analysed offline to determine particle position and angle. We confirm that the applied pressure and the flow speed remain constant throughout the course of an experiment by synthesizing a disc and tracking its motion along the channel. The flow speed is determined by tracking 1.6 μm fluorescent tracer beads mixed with the flowing solution [33] , illustrated in Supplementary Fig. S11 . For experiments presented in Fig. 7 , we synthesize fluorescent particles using CFL. To covalently bind fluorescent dye to the synthesized particles, we add acrylate-modified rhodamine to acrylate oligomer and photoinitiator solution. The synthesized particles are collected in a Tris-EDTA buffer containing 0.1 vol/vol surfactant Tween-20 in an 1.7 ml Eppendorf tube. The collected particles are resuspended in an approximately density matched solution containing 25% vol/vol poly(ethylene glycol) (molecular weight 400 g mol −1 ) in Tris-EDTA buffer. Fluorescent particles are pumped through the detection channel. Particles are imaged with an appropriate ultraviolet light source and filter set for Rhodamine. The synthesis and detection channels are 30 μm in depth, 300 μm in width and 2.4 cm in length. We have analysed over 300 symmetric and asymmetric particles. Further details regarding the experimental set-up and procedures are described in Supplementary Methods . How to cite this article: Uspal, W. E. et al. Engineering particle trajectories in microfluidic flows using particle shape. Nat. Commun. 4:2666 doi: 10.1038/ncomms3666 (2013).